Single-cell transcriptomic atlas of the human retina identifies cell types associated with age-related macular degeneration Genome-wide association studies (GWAS) have identified genetic variants associated with age-related macular degeneration (AMD), one of the leading causes of blindness in the elderly. However, it has been challenging to identify the cell types associated with AMD given the genetic complexity of the disease. Here we perform massively parallel single-cell RNA sequencing (scRNA-seq) of human retinas using two independent platforms, and report the first single-cell transcriptomic atlas of the human retina. Using a multi-resolution network-based analysis, we identify all major retinal cell types, and their corresponding gene expression signatures. Heterogeneity is observed within macroglia, suggesting that human retinal glia are more diverse than previously thought. Finally, GWAS-based enrichment analysis identifies glia, vascular cells, and cone photoreceptors to be associated with the risk of AMD. These data provide a detailed analysis of the human retina, and show how scRNA-seq can provide insight into cell types involved in complex, inflammatory genetic diseases. The human retina is a complex light-sensitive tissue that is composed of a diverse number of cell types (Fig. 1b ). Rod and cone photoreceptors convert visible light into neural signals, which are then transmitted to the brain through second-order bipolar cells and third-order ganglion cells. Horizontal and amacrine cells, two types of interneurons, provide inhibitory signals to neurons in the retina. Glial cell types include macroglia (Müller glia and astrocytes) and microglia. Among the glial cell types, Müller glia are the most common with processes that extend radially across all three retinal layers, where they provide neuronal metabolic support, supply neurotrophic factors, and maintain tissue homeostasis [1] , [2] . Prior studies of the human retina have defined cell types based on morphology, function, or the expression of a limited number of genes [3] . In contrast, single-cell RNA sequencing (scRNA-seq) allows genome-wide profiling of gene expression of thousands of cells at one time. This has previously been performed in the mouse retina and in mouse bipolar cells using Drop-seq [4] , [5] , as well as in macaque retina [6] . Fig. 1 Single-cell transcriptomic analysis reveals human retina diversity. a Study design and sample preparation. Postmortem human retinas were enzymatically dissociated and single-cells were isolated. cDNA single-cell libraries were generated and sequenced. We profiled 20,091 cells across the retinas of three normal individuals using a droplet-based microfluidics scRNA-seq platform. b Sketch of retina cross-section showing layers and major cell types. c Cell-to-cell similarity network of retinal cells. d Average expression of known cell-type marker genes across cell groups. e Projection of known cell-type-specific marker gene expression across cell groups. d , e show localization of distinct cell types within the network, identifying neighborhoods of rods, cones, retinal ganglion cells, bipolar cells, amacrine cells, horizontal cells, macroglia (Müller glia and astrocytes), microglia, and vascular cells Full size image Here, for the first time, we profile the human retina using two independent scRNA-seq platforms; droplet-based microfluidics [7] and nanowell-based Seq-Well [8] , [9] , both of which allow transcriptome-wide unbiased classification of complex tissues. We batch-correct each dataset using the mutual-nearest neighbor algorithm [10] , and construct a multiresolution cell–cell similarity network using the ACTIONet framework [11] . We consistently identify the major retinal cell types across both platforms, indicating the reproducibility of our dataand computational analysis. To explore heterogeneity within macroglial cells, both Müller glia and astrocytes, we construct an independent subACTIONet, which reveals three distinct subtypes. Finally, we use a well-established statistical framework, Multi-marker Analysis of GenoMic Annotation (MAGMA) [12] , to test the association of age-related macular degeneration (AMD) GWAS signals with specific cell types [13] , [14] , [15] , [16] . This analysis identifies potentially pathogenic cell types with preferential expression patterns predictive of AMD genetic risk. Generation of the human single-cell retinal transcriptomic atlas We isolated and sequenced retinal cells from whole retinal suspensions of the macula and periphery from six postmortem human retinas, using both the microfluidics and Seq-Well scRNA-seq platforms (Fig. 1a ). Following preprocessing and quality control (Supplementary Table 2 ), a total of 20,091 and 3,248 cells were retained for further analysis from the microfluidics and Seq-Well platforms, respectively. 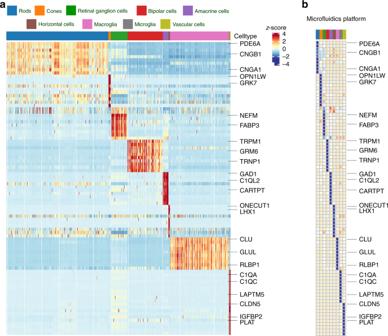Fig. 2 Heatmap of top marker genes within retinal cell types using microfluidics scRNA-seq. The top differentially expressed genes were selected using the one-sided Wilcoxon rank-sum test, and ranked based on their discriminating scores within each identified cell type.aImputed gene expression, using network diffusion, across all cells,bAverage of raw expression of each gene within each cell-type. In both panels, rows correspond to genes and columns to cell-types, which are color-coded (color bar, top) We used the mutual-nearest neighbor algorithm to correct for batch effects across different samples (Supplementary Fig. 2 ). Using a recently developed algorithm, archetypal-analysis for cell-type identification (ACTION) [11] , we extracted a set of underlying cell states, termed archetypes that explain transcriptional heterogeneity with increasing resolution. We then used our ACTION-based network (ACTIONet) framework to combine these factorizations into a multiresolution, k*-nearest neighbor graph [17] that encompasses all different levels of resolution. The ACTIONet framework couples the power of network-based analysis with the benefits of matrix decomposition techniques to analyze and visualize single-cell data. Finally, to visualize the topography of the cell space landscape, we applied a modified version of the stochastic gradient descent-based layout method used in the uniform manifold approximation and projection (UMAP) algorithm [18] using the ACTIONet graph as input (Fig. 1c ). We used a curated set of known cell-type specific markers to annotate individual cell groups. For each cell, we independently imputed the expression profile of cell-type specific markers and aggregated them into a unique score per cell type. These aggregated scores were then used to interpret and assign each cell to the most likely cell type. We observed that these independently assigned cell types localize within the cell network, defining major cell groups (Fig. 1c , Supplementary Fig. 3a ). To further verify these annotations, we projected the expression of individual markers onto the cell network (Fig. 1e , Supplementary Fig. 3c ). We found that marker expression and cell assignments partitioned the network into neighborhoods that corresponded to retinal cell types, including rod and cone photoreceptors, bipolar cells, amacrine cells, horizontal cells, microglia, retinal ganglion cells, vascular cells, Müller glia, and astrocytes. Average expression of markers across identified cell types showed high specificity, supporting the identified cell groups (Fig. 1d , Supplementary Fig. 3b ). Of note, the relative frequencies of major cell types in our data showed minor variation from earlier estimates that are potentially due to biases in sampling such as age of donor, viability of cell types, or other sample preparation variation (Supplementary Fig. 4 ). Cone photoreceptors expressed the cone-specific alpha subunit of transducin (GNAT2), and the short-wavelength (OPN1SW; blue), medium-wavelength, (OPN1MW; green), and long-wavelength (OPN1LW; red) opsins. Rod photoreceptors were distinguished based on expression of phosphodiesterase 6-alpha (PDE6A), protein phosphatase with EF-hand domain 2 (PPEF2), the nuclear receptor transcription factor (NR2E3) (Fig. 1d, e ). Retinal ganglion cells were identified based on the expression of the neurofilament medium polypeptide (NEFM) and the solute carrier family 17 member 6 (SLC17A6). Bipolar cells were marked based on expression of the marker Calcium/Calmodulin-dependent protein kinase II (CAMK2B), the glutamate metabotropic receptor 6 (GRM6), the transmembrane protein 215 (TMEM215), and the transient receptor potential cation channel subfamily M member 1 (TRPM1). Glutamate decarboxylase 1 (GAD1) and complement C1q like 2 (C1QL2) labeled amacrine cells. The transcription factors (ONECUT1, ONECUT2, and LHX1) allowed identification of horizontal cells. The cell group corresponding to Müller glia and astrocytes was identified based on expression of glutamine synthetase (GLUL), clusterin (CLU), and apolipoprotein E (APOE). The group of cells corresponding to resident microglia was identified based on the expression of complement protein (C1QA), transmembrane protein 119 (TMEM119), allograft inflammatory factor 1 (AIF1) and CD163. 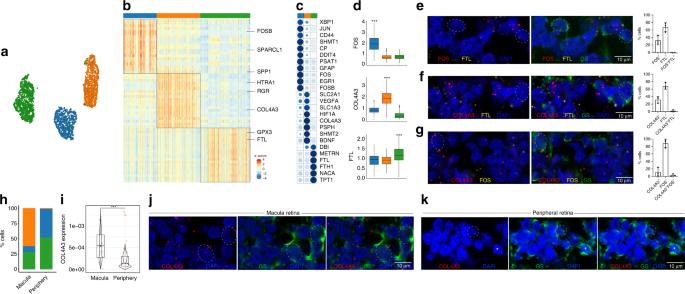Fig. 3 Heterogeneity within Müller glia and astrocytes in the human retina.aCell-to-cell similarity network (ACTIONet) representation of the filtered set of Müller glia and astrocytes, highlighting three major subtypes.bScaled heatmap of top differentially expressed genes within different cell groups.cDot plot showing the row-normalized (z-score) mean expression of the top-ranked genes across subtypes of macroglial cells.dImputed expression of key marker genes, normalized by the average of their expression across all macroglial cells. ***p< 0.001, one-sided Wilcoxon rank-sum test. Box plots are centered around the median, with the interquartile range (IQR) defining the box. The upper whisker extends to the largest value and the lower whisker extends to the smallest value, no further than 1.5 × IQR from the end of the box.e–gRepresentative images of multiplex in situ hybridization ofeFTL (labeled in yellow) and FOS (labeled in red),fFTL (labeled in yellow) and COL4A3 (labeled in red), andgFOS (labeled in yellow) and COL4A3 (labeled in red), with immunofluorescence of glutamine synthetase (GS, identified in green). Bar graphs showing frequencies ofeFOS+, FTL+, or FOS+FTL+GS+macroglia in the macula retina,fCOL4A3+, FTL+, or COL4A3+FTL+GS+macroglia in the macula retina, andgCOL4A3+, FOS+, or COL4A3+FOS+GS+macroglia in the peripheral retina. Error bars show standard error of mean. White circles indicate positive cells. Data are representative of three independent experiments.hBar graph showing frequency of each subset within the macula vs. peripheral region of the retina.iViolin plot showing gene expression differences of COL4A3 between the macula and peripheral retina. Difference is statistically significant withp< 0.01, one-sided Wilcoxon rank-sum test.j–kRepresentative images of multiplex in situ hybridization of COL4A3 (labeled in red) with immunofluorescence of glutamine synthetase (GS, identified in green) in thejmacula, andkperipheral retina. White circles indicate COL4A3+cells, and white asterisk indicates COL4A3−cells. Data is representative of three independent experiments Cells lining the retinal vasculature were marked by CD34, cadherin 5 (CDH5), Regulator Of G Protein Signaling 5 (RGS5), and the ADAM metallopeptidase with Thrombospondin Type 1 Motif 9 (ADAMTS9) (Fig. 1d, e ). Having established that our constructed network recovered known major cell types, we independently analyzed both scRNA-seq platforms to identify the top differentially expressed markers for each cell type (adjusted p -value < 0.001, one-sided Wilcoxon rank-sum test, 0.5 < area under the curve, and 0 < fold change) to identify genes with increased expression in a given cell type, relative to cells outside the group. We then selected genes that were significant in exactly one cell type, resulting in 5,504 and 7,018 differentially expressed genes for the microfluidics-based and Seq-Well platforms, respectively. For each cell type, we then ranked genes according to their cell type discriminating power score (Methods), and selected the top ten genes for visualization in both scRNA-seq platforms (Fig. 2 , Supplementary Fig. 6 ). A majority of known cell type-specific markers were observed among the set of identified top-ranked differentially expressed genes. The signature profile of each platform, as well as the one-sided Wilcoxon test results, are provided as Supplementary Tables 3 – 6 . Fig. 2 Heatmap of top marker genes within retinal cell types using microfluidics scRNA-seq. The top differentially expressed genes were selected using the one-sided Wilcoxon rank-sum test, and ranked based on their discriminating scores within each identified cell type. a Imputed gene expression, using network diffusion, across all cells, b Average of raw expression of each gene within each cell-type. In both panels, rows correspond to genes and columns to cell-types, which are color-coded (color bar, top) Full size image We then evaluated whether the list of identified marker genes, and their corresponding discriminating power, is consistent across both the microfluidics and Seq-Well platforms. Partial Pearson’s correlation analysis of archetypal cell states across platforms identified aligned major retinal cell groups, corresponding to cone and rod photoreceptors, bipolar cells, amacrine cells, horizontal cells, macroglia, microglia, vascular cells, and retinal ganglion cells (Supplementary Fig. 7 ). Overall, these results indicate that identified cell states, cell types, and differentially expressed markers are consistent across platforms, supporting the technical reproducibility of the results. Diversity of human retinal glia While the diversity of neuronal cell types in the retina is well established [19] , the complexity of macroglia in the human retina is not well-understood. Studies have shown differences in the morphology of Müller glia in the chick retina [20] , [21] , and identified Müller glia as having the capacity to generate a limited number of photoreceptor cells using gene manipulation in mice [22] ; however, little is known regarding transcriptomic heterogeneity of glia within the human retina. Closer examination of our microfluidics scRNA-seq data revealed gene expression heterogeneity within macroglia in the retina. To explore this heterogeneity, we extracted the macroglial cells, which were filtered, batch-corrected using the mutual-nearest neighbor algorithm, and used to construct a macroglia-specific cell network termed subACTIONet. This network partitioned into three distinct regions (Fig. 3a ), corresponding to putative new subtypes, which were distributed across the individual retinas (Supplementary Fig. 8a ). Using a combination of one-sided Wilcoxon rank-sum test coupled with gene discriminatory scores, we identified differentially expressed genes significantly associated with each subtype (Fig. 3b, c , Supplementary Tables 7 and 8 ). We visualized the imputed expression of the top differentially expressed genes for each subclass across all cells (Fig. 3b ). In addition, we summarized the average expression of each gene across all cells of the same subtype, to ensure reproducibility of the overall expression patterns (Fig. 3c ). Three subtype-specific markers, FOS, FTL, and COL4A3, had significantly higher expression within their corresponding subpopulation (adjusted p -value < 0.001, one-sided Wilcoxon rank-sum test) (Fig. 3d ), which we verified using fluorescent in situ hybridization. The expression patterns of ubiquitously expressed genes (GAPDH and UBC) were uniformly observed across all cells (Supplementary Fig. 8d, e ). Fig. 3 Heterogeneity within Müller glia and astrocytes in the human retina. a Cell-to-cell similarity network (ACTIONet) representation of the filtered set of Müller glia and astrocytes, highlighting three major subtypes. 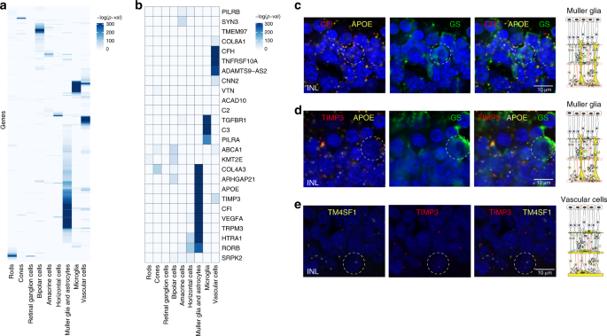Fig. 4 Cell-type specificity of AMD-associated genes using microfluidics scRNA-seq.aGene expression specificity of 585 genes previously associated with the 34 AMD locus regions defined by the 52 identified variants and their proxies (r2≥ 0.5, ±500 kb), reported in Fritsche et al.37. Specificity scores are computed using one-sided Wilcoxon rank-sum test, and reported as the log-transformed value of the adjustedp-values.bGene expression enrichment scores for the leading AMD genes, defined for each locus as the gene nearest to the lead variant (variant with smallestPvalue), as reported in Fritsche et al.37.c–eExpression pattern of AMD risk alleles CFI and TIMP3 in the human retina. Representative images of multiplex in situ hybridization with immunofluorescence ofcAPOE (labeled in yellow, identifies Müller glia), CFI (labeled in red) and glutamine synthetase (GS, identified in green);dAPOE (labeled in yellow, identifies Müller glia), TIMP3 (labeled in red) and glutamine synthetase (GS, identified in green), andeTM4SF1 (labeled in yellow, identifies vascular endothelium) and TIMP3 (labeled in red). White dotted circles indicate double positive cells. Data are representative of three independent experiments 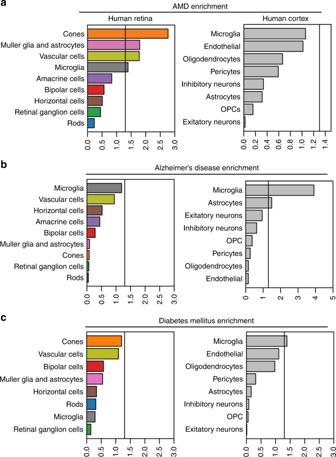Fig. 5 Cell-type trait association analyses. Bars show the mean strength of association computed with MAGMA (-log10P) for AMD (a) Alzheimer’s Disease (b), and Diabetes Mellitus (c) using cell type preferential gene expression in either the human retina microfluidics scRNA-seq dataset (left) or the human cortex scRNA-seq dataset as a control (right). The vertical line indicates whether the cell-type is significantly associated with the trait (P< 0.05, MAGMA gene-set analysis test, linear regression) b Scaled heatmap of top differentially expressed genes within different cell groups. c Dot plot showing the row-normalized ( z -score) mean expression of the top-ranked genes across subtypes of macroglial cells. d Imputed expression of key marker genes, normalized by the average of their expression across all macroglial cells. *** p < 0.001, one-sided Wilcoxon rank-sum test. Box plots are centered around the median, with the interquartile range (IQR) defining the box. The upper whisker extends to the largest value and the lower whisker extends to the smallest value, no further than 1.5 × IQR from the end of the box. e – g Representative images of multiplex in situ hybridization of e FTL (labeled in yellow) and FOS (labeled in red), f FTL (labeled in yellow) and COL4A3 (labeled in red), and g FOS (labeled in yellow) and COL4A3 (labeled in red), with immunofluorescence of glutamine synthetase (GS, identified in green). Bar graphs showing frequencies of e FOS + , FTL + , or FOS + FTL + GS + macroglia in the macula retina, f COL4A3 + , FTL + , or COL4A3 + FTL + GS + macroglia in the macula retina, and g COL4A3 + , FOS + , or COL4A3 + FOS + GS + macroglia in the peripheral retina. Error bars show standard error of mean. White circles indicate positive cells. Data are representative of three independent experiments. h Bar graph showing frequency of each subset within the macula vs. peripheral region of the retina. i Violin plot showing gene expression differences of COL4A3 between the macula and peripheral retina. Difference is statistically significant with p < 0.01, one-sided Wilcoxon rank-sum test. j – k Representative images of multiplex in situ hybridization of COL4A3 (labeled in red) with immunofluorescence of glutamine synthetase (GS, identified in green) in the j macula, and k peripheral retina. White circles indicate COL4A3 + cells, and white asterisk indicates COL4A3 − cells. Data is representative of three independent experiments Full size image The first subtype (FOS-expressing) was enriched with markers known to be expressed in astrocytes including intermediate-filament glial fibrillary acidic protein (GFAP) and the sparc-like protein (SPARCL1) [5] , [23] . Within this subtype, the immediate-early response genes FOS, FOSB, JUN, and EGR1 [24] were also detected (Fig. 3c ). While we cannot exclude the possibility that this subtype represents Müller glia that have undergone reactive gliosis [25] , it would be more consistent with astrocytes, as this subtype was observed across all retinas with no known pathology. Furthermore, this subtype was found to be significantly enriched in the periphery of the retina, compared to the macula ( p -value < 0.001, one-sided Wilcoxon rank-sum test) (Supplementary Fig. 8c ). This is in agreement with previous studies reporting that CD44 and EGR1, two genes enriched within this subtype, are expressed highly in the peripheral retinal regions [26] , [27] . It is also consistent with the regional localization of astrocytes within the human retina [28] . The second subtype displayed increased expression of multiple genes associated with AMD including COL4A3, vascular endothelial growth factor (VEGFA), and HTRA1, and was found to be significantly enriched in the macula compared to the periphery (Fig. 3h–k ). COL4A3 is a gene linked to Alport Syndrome, where a majority of patients frequently develop a maculopathy [29] , further supporting a role for this subset in regional-susceptibility of disease. Furthermore, significant upregulation of genes associated with metabolism including the glucose transporter (SLC2A1/GLUT1), the glutamate transporter (SLC1A3/GLAST1), and Serine Hydroxymethyltransferase 2 (SHMT2), which is involved in de novo serine synthesis [30] , [31] was observed in this subset of Müller glia. Of note, GLUT1 and VEGFA are target genes of hypoxia-inducible factor HIF1A [32] , which was also found to be upregulated in this subset Fig. 3b, c ). The third subtype expressed higher levels of ferritin heavy chain (FTH1) and ferritin light chain (FTL) (Fig. 3c ). These proteins have a central role in iron homeostasis, where they bind iron and prevent its ability to cause oxidative damage to cells in the retina. Loss of Müller glia causes accumulation of iron in the retina [33] and is associated with AMD [34] , [35] , therefore highlighting a role for this subset in regulating iron levels. In addition, this macroglial subset also expresses diazepam-binding inhibitor (DBI), which regulates activation of microglia by limiting the magnitude of inflammatory responses upon initiation and facilitating a return to baseline homeostasis [36] . Given the central iron homeostasis gene signature of this subpopulation, and its ability to regulate microglial activation, further investigation will reveal whether dysfunction of this subset of macroglia contributes to accumulation of iron in the retina, oxidative damage, inflammation, and AMD pathophysiology. Of note, this FTL-expressing subset was found to be evenly distributed between the macula and peripheral regions of the retina (Fig. 3h , Supplementary Fig. 8b ). We used immunofluorescence with GS to reliably identify Müller Glia and astrocytes, in combination with FOS, COL4A3, and FTL to validate the three distinct macroglial subsets in the human retina (Fig. 3e–g ). We found that very few cells co-expressed the subset-specific genes. Furthermore, we validated the existence of distinct macroglial subsets using the independent Seq-Well scRNA-seq dataset, and found consistency of gene expression between the three subtypes (Supplementary Fig. 9 ). Moreover, to show that the identified subpopulations do not merely reflect potential, context-specific activation states in human, we analyzed the macroglial cells from the non-human primate retinal atlas from Peng et al. [6] . We found the gene signatures reported here in humans segregate three consistent subpopulations in the non-human primate retina, providing support for the conservation and robustness of the subgroups. (Supplementary Fig. 10 ). Together, these results support the existence of glial diversity in the human retina. Cell-type specific expression of AMD-associated risk loci Population-based GWAS studies have reproducibly linked genetic variants to complex diseases; however, translating these data to biological cellular mechanisms has been limited by the large number of variants associated with disease, each of which have a small effect size. In 2016, a large GWAS study (sample size > 15,000) identified 34 risk loci associated with AMD at genome-wide significance [37] . Here we used our single-cell transcriptomic retinal atlas to relate the patterns of AMD genetic risk with patterns of cell-type specific expression. First we analyzed the patterns of preferential activity of genes surrounding the 34 risk loci ( n = 585 genes, after matching with the atlas) (Fig. 4a ). All 585 genes were retained in both platforms, and have been used for our study. We found that the highest percentage of associated cells in both platforms were associated with Müller glia and astrocytes ( p- value < 1e-10, one-sided Wilcoxon rank-sum test Supplementary Fig. 12 ). Similar pattern was observed among the leading AMD-associated genes (nearest gene to lead GWAS variant), including CFI, TIMP3, VEGFA and COL4A3 (Fig. 4b ). Preferential expression scores are reported in Supplementary Tables 9 – 12 . Fig. 4 Cell-type specificity of AMD-associated genes using microfluidics scRNA-seq. a Gene expression specificity of 585 genes previously associated with the 34 AMD locus regions defined by the 52 identified variants and their proxies ( r 2 ≥ 0.5, ±500 kb), reported in Fritsche et al. [37] . Specificity scores are computed using one-sided Wilcoxon rank-sum test, and reported as the log-transformed value of the adjusted p -values. b Gene expression enrichment scores for the leading AMD genes, defined for each locus as the gene nearest to the lead variant (variant with smallest P value), as reported in Fritsche et al. [37] . c – e Expression pattern of AMD risk alleles CFI and TIMP3 in the human retina. Representative images of multiplex in situ hybridization with immunofluorescence of c APOE (labeled in yellow, identifies Müller glia), CFI (labeled in red) and glutamine synthetase (GS, identified in green); d APOE (labeled in yellow, identifies Müller glia), TIMP3 (labeled in red) and glutamine synthetase (GS, identified in green), and e TM4SF1 (labeled in yellow, identifies vascular endothelium) and TIMP3 (labeled in red). White dotted circles indicate double positive cells. Data are representative of three independent experiments Full size image We validated the cell type preferential expression of a subset of AMD-associated genes with fluorescent in situ hybridization. Tissue inhibitor of metalloproteinase 3 (TIMP3) is an extracellular protein deposited in the extracellular matrix, where it inhibits retinal neovascularization through blocking the vascular endothelial growth factor receptor-2 [38] and matrix metalloproteinases [39] . We validated that TIMP3 is expressed in Müller glia through co-localization with APOE, and in vascular cells through co-localization with TM4SF1 (Fig. 4d, e ), in addition to its previously reported expression in the retinal pigment epithelium [39] . Complement factor I is a serine protease that proteolytically cleaves C3b inhibiting activation of the alternative complement pathway. This complement factor co-localized with APOE in Müller glia, among other retinal cell types (Fig. 4c ). Cell-type specific associations of AMD genetic risk To determine whether the patterns of preferential expression are predictive of genetic risk, and in particular, to identify the cell types whose gene signatures correlate the most with genetic risk, we used MAGMA [12] , [15] . For this analysis, we considered the set of genes preferentially expressed in each cell type (one-sided Wilcoxon rank-sum test, FDR < 0.01 and detected in at least 25% of the cells in the group). We identified that cone photoreceptors, macroglia, microglia, and vascular cells are the most predictive of AMD risk (Fig. 5a ). We confirmed that the same pattern of association does not occur when considering cell type expression specificity, within the scRNA-Seq of the human cortex [40] (Fig. 5a ). We also confirmed that the cell types and gene signatures identified in our retinal atlas are not similarly predictive of genetic risk when considering other traits, using Alzheimer’s disease [41] and Diabetes mellitus [42] as negative controls (Fig. 5b, c ). Together, our data provide a framework to identify cell types that are likely to be more vulnerable to genetic perturbations and influence AMD susceptibility. Fig. 5 Cell-type trait association analyses. Bars show the mean strength of association computed with MAGMA (-log10P) for AMD ( a ) Alzheimer’s Disease ( b ), and Diabetes Mellitus ( c ) using cell type preferential gene expression in either the human retina microfluidics scRNA-seq dataset (left) or the human cortex scRNA-seq dataset as a control (right). The vertical line indicates whether the cell-type is significantly associated with the trait ( P < 0.05, MAGMA gene-set analysis test, linear regression) Full size image It was previously thought that AMD was due to pathology of the photoreceptors and retinal pigment epithelium [39] . While our results demonstrate that the genetic risk variants contributing to AMD affect cone photoreceptors, they are associated with additional cell types, highlighting the importance of glial and vascular cells in disease pathogenesis. Patients with neovascular AMD develop pathological angiogenesis and fibrosis, which is supported by our finding of significant association of AMD risk genes with macroglia, microglia, and vascular cells in the human retina. Based on our single-cell transcriptomic atlas, our data predicts that these cell types preferentially contribute to the pathogenesis of AMD, and provide genetic context to target these cell types for the development of new disease therapies. 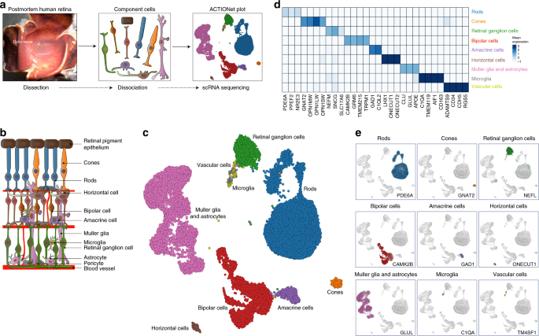In summary, our results provide a reference single-cell atlas of the adult human retina. We identify unexpected gene expression heterogeneity of macroglia in the retina, suggesting that human retinal glia are more diverse than previously thought. Our retinal atlas gives insight into AMD pathogenesis, and identifies cone photoreceptors, glial, and vascular cell types, in which the genetic risk can be traced. This retinal cell atlas will enhance our knowledge of normal retinal biology as well as disease pathogenesis. Fig. 1 Single-cell transcriptomic analysis reveals human retina diversity.aStudy design and sample preparation. Postmortem human retinas were enzymatically dissociated and single-cells were isolated. cDNA single-cell libraries were generated and sequenced. We profiled 20,091 cells across the retinas of three normal individuals using a droplet-based microfluidics scRNA-seq platform.bSketch of retina cross-section showing layers and major cell types.cCell-to-cell similarity network of retinal cells.dAverage expression of known cell-type marker genes across cell groups.eProjection of known cell-type-specific marker gene expression across cell groups.d,eshow localization of distinct cell types within the network, identifying neighborhoods of rods, cones, retinal ganglion cells, bipolar cells, amacrine cells, horizontal cells, macroglia (Müller glia and astrocytes), microglia, and vascular cells Human tissues Postmortem eyes for the Chromium Single Cell 3′ assay ( n = 3) and dual RNAscope/Immunofluorescence experiments ( n = 2) were procured from Alabama Eye Bank with a maximum processing time of 3.5 h (Supplementary Table 1 ). Postmortem eyes for the Seq-Well single-cell RNA-seq platform ( n = 3) and RNAscope ( n = 2) were collected from autopsies at Massachusetts General Hospital (Boston, MA) with an average processing time of 17 h. Eyes were collected from August 2017 through March 2019. Globes were examined for retinal disease by an ophthalmologist (B.P.H) prior to dissection and dissociation of the samples. Retinas collected for this study had no known retinal disease and no abnormalities indicative of disease pathology. This study was approved by the Partners Institutional Review Board. We complied with all relevant ethical regulations for work with human participants, and informed consent was obtained. Retinal dissection and dissociation Globes were placed in Dulbecco’s Modified Eagle Medium media (ThermoFisher) and transported on ice. Trephine punches (6 mm diameter) were used to isolate samples from (1) the macula in the central retina and (2) a region of mid-peripheral retina, located away from the optic disc and major arterioles. For each punch of tissue, the retina was mechanically separated from the underlying retinal pigment epithelium-choroid. Retinal and RPE-choroid layers were processed separately during dissociation. The remaining tissue was snap-frozen on dry ice and stored at −80 °C for RNA quality metrics and validation experiments. Retinal samples were processed using a single-use papain dissociation system (Worthington, Catalog No. LK003150). Briefly, the retinal samples were minced with scalpels and dissociated by incubation with a buffer containing papain (20 U/ml) supplemented with DNAse-I (2000 U/ml) in Earle’s Balanced Salt Solution at 37 °C for 30 min in an incubator with end-over-end rotation. Samples were triturated 15 times with a 5-mL serological pipette and the dissociation process was ended with the addition of the protease inhibitor, ovomucoid. Cell suspensions were passed through a single step discontinuous density gradient, resuspended in Earle’s Balanced Salt Solution with 10% Fetal Bovine Serum and passed through a 100-µm nylon cell strainer. The final cell suspensions were counted with trypan blue for viability prior to loading on the single-cell platform. Samples on average displayed 90% viability. Droplet-based microfluids scRNA-seq Single-cell libraries were prepared using the Chromium 3′ v3 platform (10X Genomics) following the manufacturer’s protocol. Briefly, single cells were partitioned into Gel beads in Emulsion in the 10X Chromium Controller instrument followed by cell lysis and barcoded reverse transcription of RNA, amplification, shearing and 5′ adapter and sample index attachment. On average, ~7000 cells were loaded on each channel that resulted in the recovery of ~4000 cells. Libraries were sequenced on Illumina NextSeq 500, Paired end reads: Read 1, 26 bp, Read 2, 98 bp. Seq-Well scRNA-seq A total of 10,000 freshly dissociated retinal cells were loaded on each Seq-Well array preloaded with barcoded mRNA capture beads (ChemGenes) [8] . Seq-Well used a polydimethylsiloxane (PDMS) array of ~86,000 subnanoliter wells. The loaded arrays were then sealed with a polycarbonate membrane (Sterlitech 0.01 µm pore size, 62 × 22 mm), which allowed buffer exchange while retaining biological molecules within nanowells. Cells were pre-lysed with 5 M Guanidine thiocyanate (Sigma) and 1 mM EDTA (Sigma), then lysed with 5 M Guanidine thiocyanate, 1 mM EDTA, 0.50% Sarkosyl (Sigma), and 1.0% 2-Mercaptoethanol (Sigma), and transcripts were hybridized to the mRNA capture beads. The polycarbonate membrane was removed, the beads collected, and reverse transcription performed in bulk using Maxima H Minus Reverse Transcriptase (ThermoFisher EP0753). Exonuclease I (NewEngland Biolabs M0293L) was used to degrade excess primers. PCR amplification was performed using KAPA HiFi PCR Mastermix (Kapa Biosystems KK2602) with 2,000 beads per 50 µL reaction volume and the Smart PCR primer AAGCAGTGGTATCAACGCAGAGT. Each sample generated ~12 PCR reactions. Six libraries (comprised of ~12,000 beads) were pooled together and purified with Agencourt AMPure XP beads (Beckman Coulter, A58581), once with a 0.7X AMPure SPRI volumetric ratio followed by a 0.9X AMPure SPRI ratio. Library quantification was determined with the Qubit dsDNA HS Assay (ThermoFisher Q32854). Libraries were constructed using 800 pg of pooled cDNA product and the Nextera XT Library kit. Samples were barcoded with Nextera N700 indices, one per library [8] . Final library products were purified with 0.6X AMPure SPRI ratio, determined using the Agilent High Sensitivity D1000 ScreenTape system (Agilent Genomics). Arrays were sequenced with Illumina NextSeq 500. Data preprocessing Sample demultiplexing, read alignment to the NCBI reference genome, quantification and initial quality control (QC) of the microfluidics-based sequencing dataset was performed using the Cell Ranger Software (version 3.0.2; 10X Genomics) for each sample separately. We used the option “-forcecells 4000” in Cell Ranger count to extract a larger number of cell barcodes in the data, as the automatic estimate by Cell Ranger was too conservative as previously reported (Peng et al. [6] ). We grouped the count matrices from 6 samples, and prefiltered to include only cells that have at least 300 genes (with each gene expressed by a minimum of 10 cells) for further analysis to generate a 19,719 genes × 20,091 cell matrix for further analysis. Read alignment of the Seq-Well-based sequencing dataset was performed mostly as described in Macosko et al. [5] Briefly, raw sequencing runs were converted to demultiplexed FASTQ files using bcl2fastq2 based on the Nextera N700 indices denoted above. FASTQ files were then aligned to the hg19 genome using standard settings for the Drop-Seq alignment on the Galaxy portal (Broad Institute) using the STAR aligner. Finally, we prefiltered count matrices to include only cells that have at least 300 identified transcripts and genes that are expressed in at least 10 cells, and generated a 18,219 genes × 3,248 cell matrix for further analysis. Potential cross-sample batch effects were corrected for using the mutual-nearest neighbor method [10] . Cell state characterization ACTIONet framework ( https://github.com/shmohammadi86/ ACTIONet) was used to identify cell types/states, as well as to construct an adaptive, multiresolution network of cell–cell similarities. In summary, multiple independent ACTION-based factorizations [11] with increasing number of archetypes (underlying cell state patterns) are performed, and the corresponding archetypes are used to define a metric space that represent pairwise similarity among cells, measured using the square-root of the Jensen-Shannon divergence. A k-adaptive nearest neighbor similarity network was then constructed within this space using the k*-nearest neighbors algorithm, which selects the optimal number of neighbors at each node based on the distance between the neighbors [17] . In this view, ACTIONet can be seen as a compressed network representation that encapsulates multiple archetypal analysis-based matrix decompositions. The resulting network was used throughout the study to visualize, characterize, and interactively explore the transcriptional cell state space. Supplementary Fig. 3 shows the frequency of human retinal cell types identified using both microfluidics and Seq-Well sequencing platforms. Cell annotation and doublet prediction Following best practice recommendations [43] , we transformed raw count data through normalization based on count depth. A permissive quality control (QC) step was performed, followed by downstream analysis using the ACTIONet framework. Additional, putative low-quality cells were filtered out after post-processing as needed. More specifically, a manually curated set of marker genes encompassing all known major cell types in the retina was used to assess the putative identity of each cell. The value of each marker gene was imputed across all cells using a diffusion-based algorithm, and then individual markers corresponding to a given cell type were aggregated into a cell type-association score computed per each cell. A permutation test was subsequently used to assess the deviation from expectation of observed association scores. Cells that were either (i) not significantly associated with any cell type, or (ii) were significantly associated with more than one cell type, were filtered out from our study, due to the suspicion of potential doublets. Evidence of low quality of cells was additionally suggested by their isolated positioning in the network with respect to other highly clustering cells. For the rest of the cells, the cell type with the highest association score was selected as the most likely cell type annotation. Finally, the network context was used to filter out cells that were annotated with a given cell type, but their respective network neighbor cells were not statistically enriched with that same cell type annotation. We assume that such cells likely correspond to technical artifacts, such as doublets. For the macroglia cell subnetwork, cells marked as microglia were extracted and independently analyzed with the ACTIONet framework. Prior to analysis, mutual-nearest neighbor was used again for batch correction to remove residual batch effects, and a subset of cells simultaneously expressing both macroglial and rod-specific markers potentially representing doublets was removed. Identification of top differentially expressed genes To identify de novo markers, we first constructed a signature profile for each cell type in each platform, independently. More specifically, we combined the PCA-reduced profile of cells, after the ACTION-preprocessing step [11] , within each cluster to have an aggregate profile of meta-genes, one per each cluster. Then, we applied a linear-transformation using the left-singular vectors of the expression matrix to transform “ metagene x cell type” matrix back to the “ gene x cell type” . These cell type signature profiles measure the influence of each gene in distinguishing one cell type from the rest–or their discriminating power . However, these genes can still be shared across groups of related cell types, for example pan-neuronal genes among neuronal cell types. To further prune this set, we used the one-sided Wilcoxon rank-sum test and selected genes that are significant for one cell type. To evaluate the consistency of the signature profile of genes within different cell types across platforms, we computed the pairwise partial Pearson’s correlation between pairs of cell type-specific signature vectors between microfluidics and Seqwell platforms, respectively; after controlling for the baseline discriminatory power of genes across cell types in each platform. Among computed correlations, retinal ganglion cells had the lowest matching rate, while bipolar cells, rods and macroglial cells showed the highest overlap. which has been attributed to the rod-gene contamination in the 10X dataset. Dissecting heterogeneity of macroglial cells We first extracted the cells annotated as macroglial in the first round (main ACTIONet) and created a new count matrix. We then batch corrected this count matrix, reduced it using the ACTION kernel, and reconstructed a subACTIONet for macroglial cells. Upon annotation, we have found macroglial cells that were further contaminated with the rod markers, and filtered them from our study. The final macroglial subACTIONet contained 2,537 filtered/batch-corrected macroglial cells, which formed three distinct clusters. We have analyzed each cluster, and reported their corresponding markers. Cell-type-specific enrichment of AMD-associated genes The set of genes surrounding the the 34 AMD locus regions (defined by the 52 identified variants and their proxies ( r 2 ≥ 0.5, ±500 kb) were obtained from the genome-wide association study [37] . Among these genes, a total of 585 genes mapped to genes in the scRNA dataset after QC, which we used as a proxy to analyze cell type-specificity of AMD-associated genes. For each gene, we used one-sided Wilcoxon rank-sum test to assess its specificity within each cell type, and used log-transformed adjusted p- values as a measure of cell type specificity. We set p -values smaller than 1e-300 to 1e-300 (to avoid Inf log-scores), and set a stringent p -value significance threshold of 1e-10. Association between genes preferentially expressed in a given cell type and AMD genetic risk scores was performed using MAGMA [12] , testing for a positive correlation between cell type expression specificity and gene-level GWAS-based genetic associations scores. For this analysis genes with increased expression in a given cell type relative to other cells (one-sided Wilcoxon rank-sum test, FDR < 0.01) and which are detected in at least 25% of the cells in the group were considered as gene sets. The GWAS summary statistics [37] , [41] , [42] and scRNA-Seq of the human cortex [40] reported in previous studies were used. All GWAS summary statistics datasets were downloaded from the GWAS Atlas ( https://atlas.ctglab.nl/ ). In situ hybridization Posterior poles were fixed in 4% paraformaldehyde in PBS at 4 °C for 12 h and passed through 10, 20, and 30% sucrose gradients prior to embedding in optimum cutting temperature compound (OCT). Sections were air-dried at −20 °C for 12 h and moved to −80 °C for long-term storage. In situ hybridization was performed on 10 µm tissue sections using the RNAScope Multiplex Fluorescent v2 Assay , with minor modifications to the manufacturer’s recommended protocol. Specifically, OCT was removed by incubation with 1X PBS for 3 min at room temperature (RT). Slides were then baked in an oven for 45 min at 60 °C, and fixed in 10% neutral-buffered formalin for 90 min at RT. Slides were dehydrated with four ethanol gradients (50%, 70%, 100%, 100%), and hydrophobic barriers were applied (Immedge PAP Pen, Cat No. H-4000). Antigen retrieval consisted of hydrogen peroxide for 10 min at RT, followed by protease III for 30 min at 40 °C. Following probe hybridization, slides were washed with RNAScope Wash Buffer, and stored overnight in 5X SSC at RT. The probes used include COL4A3, APOE, FOS, FTL, CFI, TIMP3, and TM4SF1 . Following the assay, slides were stained with glutamine synthetase (GS) in a 1:500 dilution (BD Biosciences, 610518), as recommended in the RNAScope Combined Immunofluorescence technical note. A positive cell was defined based on the expression of one or more positive spots. The co-expression of two genes in a cell was determined by automated fluorescence analysis using FIJI/ImageJ (ImageJ macro available upon request), and counts verified manually. The positive control probes RNA polymerase II (POLR2A) and ubiquitin C (UBC) were used to confirm RNA quality in tissue sections (Supplementary Fig. 11a ). The negative control probe, DapB from the Bacillus subtilis bacterial strain, was used to assess for background signal (Supplementary Fig. 11b ). Reporting summary Further information on research design is available in the Nature Research Reporting Summary linked to this article.